A synthetic sex ratio distortion system for the control of the human malaria mosquito It has been theorized that inducing extreme reproductive sex ratios could be a method to suppress or eliminate pest populations. Limited knowledge about the genetic makeup and mode of action of naturally occurring sex distorters and the prevalence of co-evolving suppressors has hampered their use for control. Here we generate a synthetic sex distortion system by exploiting the specificity of the homing endonuclease I-PpoI, which is able to selectively cleave ribosomal gene sequences of the malaria vector Anopheles gambiae that are located exclusively on the mosquito’s X chromosome. We combine structure-based protein engineering and molecular genetics to restrict the activity of the potentially toxic endonuclease to spermatogenesis. Shredding of the paternal X chromosome prevents it from being transmitted to the next generation, resulting in fully fertile mosquito strains that produce >95% male offspring. We demonstrate that distorter male mosquitoes can efficiently suppress caged wild-type mosquito populations, providing the foundation for a new class of genetic vector control strategies. In most pest species, males contribute few material resources to the next generation, and it is the number and productivity of females that determines future population size. The induction of extreme male-biased reproductive sex ratios has thus been suggested as an attractive method to suppress or eliminate pest populations [1] , [2] . For this reason, the identification of naturally occurring sex ratio distorters found in two medically important genera of mosquitoes, Aedes and Culex , has generated substantial interest [3] , [4] . However, attempts to assess the suitability of such natural distorter strains for controlling caged mosquito populations revealed that the degree of distortion was insufficient to achieve population suppression [5] . Resistance in female mosquitoes was often swiftly selected for, indicating the prevalence of natural resistance alleles. Although a detailed molecular understanding of these distorters has remained elusive, cytological observations indicated that a bias towards male gamete production in Aedes is associated with preferential breakage of the X chromosome during male meiosis, thus suggesting one possible mechanism of action [6] . We therefore hypothesized that the selective induction of DNA double-stranded breaks in the X chromosome during male meiosis might be a potential strategy to distort the sex ratio of the progeny towards male mosquitoes, if the normal production of Y-bearing gametes was unaffected ( Fig. 1a ). 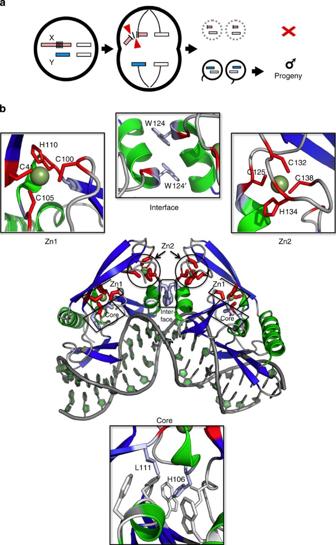Figure 1: Generation of a synthetic sex distortion system. (a) Proposed model for the distortion of the reproductive sex ratio towards males based on meiotic X shredding. A multicopy target sequence (black bars) on the X chromosome (but not present on the Y chromosome) is targeted by an endonuclease (red triangle) during spermatogenesis. Shredding of the X chromosome favours the unaffected Y-bearing sperm and results in the production of a male-biased progeny. (b) Structure of I-PpoI a homodimeric, ‘His-Cys box’ homing endonuclease that recognizes and cleaves a highly conserved rDNA sequence. Boxes: a total of 11 residues were mutated in this study. Eight of those positions correspond to residues that coordinate two zinc ions in each subunit (‘Zn1’ and ‘Zn2’). One position contributes two symmetry-related tryptophan side chains (W124 and W124′) that form a significant fraction of the dimer interface; the final two positions (L111 and H106) are found in small hydrophobic core regions in each subunit. Figure 1: Generation of a synthetic sex distortion system. ( a ) Proposed model for the distortion of the reproductive sex ratio towards males based on meiotic X shredding. A multicopy target sequence (black bars) on the X chromosome (but not present on the Y chromosome) is targeted by an endonuclease (red triangle) during spermatogenesis. Shredding of the X chromosome favours the unaffected Y-bearing sperm and results in the production of a male-biased progeny. ( b ) Structure of I-PpoI a homodimeric, ‘His-Cys box’ homing endonuclease that recognizes and cleaves a highly conserved rDNA sequence. Boxes: a total of 11 residues were mutated in this study. Eight of those positions correspond to residues that coordinate two zinc ions in each subunit (‘Zn1’ and ‘Zn2’). One position contributes two symmetry-related tryptophan side chains (W124 and W124′) that form a significant fraction of the dimer interface; the final two positions (L111 and H106) are found in small hydrophobic core regions in each subunit. Full size image Anopheles gambiae , the main vector of human malaria represents an ideal experimental model to test this hypothesis because of the availability of the highly specific homing endonuclease I-PpoI [7] , which cuts a conserved sequence within the ribosomal rDNA repeats located in a single cluster on the mosquito’s X chromosome [8] . The expression of wild-type I-PpoI during spermatogenesis in transgenic mosquitoes causes cleavage of the paternal X chromosome but also results in complete male sterility because the protein’s stability and persistence in mature sperm cells leads to subsequent cleavage of the maternal X chromosome in the zygote [9] . However, these preliminary experiments also indicated that the majority of developmentally arrested embryos had been fertilized by Y-bearing spermatozoa, providing a rationale for attempting to uncouple chromosomal transmission distortion from male sterility [9] . In this study, we systematically destabilize the I-PpoI endonuclease with the objective to reduce its in vivo half-life and thereby restrict its activity to male meiosis, which occurs earlier than the formation of the zygote after female fertilization. Our objective is population suppression via the development of transgenic male mosquitoes that are not sterile and produce mainly Y chromosome-bearing sperm (and hence will produce only male progeny when mated with wild-type female mosquitoes). Male transgenic progeny fathered by these transgenic male mosquitoes also produce Y-biased sperm so that the effect can be self-sustaining. Generation of destabilized I-PpoI variants We have generated a series of I-PpoI variants that displays a range of thermal unfolding temperatures spanning about 20 degrees, and a corresponding range of half-lives that differ by as much as 30-fold. To accomplish this, we used the crystal structure of the enzyme bound to its DNA target site to guide the necessary alterations of the protein’s sequence and structure [7] . We selected residues for site-directed mutagenesis that were involved either (i) in the coordination of structural zinc ions in the protein core, (ii) in hydrophobic packing in the protein core or (iii) in subunit interactions within the protein dimer interface ( Fig. 1b ). Of the 11 residues that were subjected to point mutagenesis, alteration of each of the eight individual residues involved in zinc coordination resulted in a dramatic reduction in expression and recovery of recombinant protein, presumably because of disrupted folding. In contrast, mutation of two residues in the hydrophobic core (H106 and L111) and one residue in the dimer interface (W124) yielded soluble proteins that were readily purified using the same protocol used for the wild-type protein (as did simultaneous mutation of L111 and W124 to alanine and leucine, respectively). The thermal denaturation temperatures (‘Tm’) of the wild-type and mutant I-PpoI proteins were then determined by conducting temperature-dependent protein denaturation experiments using circular dichroism (CD) spectroscopy on purified protein samples ( Supplementary Fig. 1a ). Under these experimental conditions the Tm of the wild-type protein was determined to be 54.4 °C (±0.2 °C). Mutations of the residues in the hydrophobic core and/or dimer interface all reduced the thermostability of the corresponding recombinant proteins with Tm values ranging from 49.4 °C (L111A; Δ T m=−5°) to 35.1 °C (L111A/W124L; Δ T m=−19.3°) while maintaining cooperative unfolding transitions for each endonuclease variant. In vitro characterization of I-PpoI variants We next performed kinetic unfolding experiments in which purified enzymes were placed at constant temperatures (30 or 37 °C) while monitoring the gradual unfolding of the protein by measuring the CD signal (sensitive to a protein’s secondary structure) at 206 nm for 4 h ( Supplementary Fig. 1b,c ). The thermal half-life of each construct at 37° ranged from 73.5 h (wild-type enzyme) to 2 h (H106A; the L111A/W124L double mutant displayed a half-life of ~4 min). At 30 °C, none of the constructs exhibited significant thermal unfolding over 4 h (except for the double mutant, which displayed a half-life of ~35–40 min). The specific activity of the wild-type and mutant enzymes was then determined using freshly prepared enzyme under assay conditions (a DNA digest performed at 22 °C for 5 min) where unfolding of each enzyme variant would not contribute to reduced catalytic activity ( Supplementary Fig. 1d,e ). With the exception of the double mutant, all of the constructs fell within a threefold activity range (from a value of ~7 pmol min −1 μg −1 for the wild-type enzyme to 2.6 pmol min −1 μg −1 for the H106A construct). The properties of all mutants are summarized in Table 1 . Table 1 Properties of wild-type and mutant I-PpoI variants determined in vitro . Full size table Generation and characterization of transgenic lines We then designed germline transformation constructs to express each of the I-PpoI structural variants showing reduced stability in transgenic mosquitoes using the male spermatogenesis-specific β2 tubulin promoter [10] ( Fig. 2a ). The constructs were designed to express both I-PpoI and enhanced green fluorescent protein (eGFP) as in frame fusion proteins or, using a 2A ribosomal stuttering signal, as distinct protein chains. We generated at least two independent transgenic lines for each I-PpoI variant. We determined the genomic location ( Supplementary Table 1 ) and I-PpoI mRNA expression levels ( Supplementary Fig. 2 ) in all transgenic lines that showed a single chromosomal integration of the transgene. Constructs that had integrated on the X chromosome failed to show significant levels of I-PpoI expression in the testes, in agreement with the notion that this chromosome undergoes general transcriptional silencing during male meiosis [11] . The mRNA abundance of strains carrying autosomally integrated constructs ranged from twofold higher to 35-fold lower compared with mosquitoes expressing wild-type I-PpoI, thus offering the possibility to assess different combinations of expression levels and thermostability. We analysed protein levels of recombinant I-PpoI in testes with western blot experiments using, for each variant, the strain with the highest level of mRNA expression. We observed that a reduced in vitro thermostability of the I-PpoI mutants translated into significantly reduced protein levels of the eGFP::I-PpoI protein variants in vivo consistent with lower eGFP fluorescence signal observed in the testes of these lines ( Supplementary Fig. 3 ). 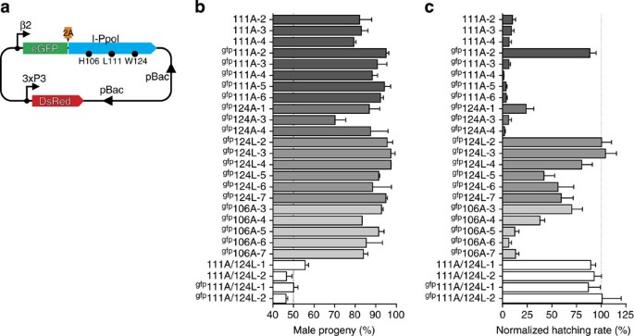Figure 2: Engineered I-PpoI variants distort the sex ratio towards males. (a) Germline transformation construct showing mutated I-PpoI residues. (pBac) piggyBac inverted repeats; (3xP3) Pax promoter driving the DsRed marker gene (DsRed); I-PpoI and GFP reading frames under the control of β2 tubulin promoter (β2); (2A) self-cleaving peptide used in some constructs. (b) The adult sex ratio (error bars represent the s.e.m.) of the progeny of hemizygous transgenic males and wild-type females of all transgenic lines with single copy autosomal integrations. Experiments were performed in at least two independent generations. The total numbers of sexed individuals are summarized inSupplementary Table 2. (c) The larval hatching rate (error bars represent s.e.m.) of the progeny of hemizygous transgenic males and wild-type females of all transgenic lines with single copy autosomal integrations normalized against the hatching rate of hemizygous transgenic females and wild-type males of the same lines. Experiments were performed in at least two independent generations. The total number of females analysed is summarized inSupplementary Table 2. Figure 2: Engineered I-PpoI variants distort the sex ratio towards males. ( a ) Germline transformation construct showing mutated I-PpoI residues. (pBac) piggyBac inverted repeats; (3xP3) Pax promoter driving the DsRed marker gene (DsRed); I-PpoI and GFP reading frames under the control of β2 tubulin promoter (β2); (2A) self-cleaving peptide used in some constructs. ( b ) The adult sex ratio (error bars represent the s.e.m.) of the progeny of hemizygous transgenic males and wild-type females of all transgenic lines with single copy autosomal integrations. Experiments were performed in at least two independent generations. The total numbers of sexed individuals are summarized in Supplementary Table 2 . ( c ) The larval hatching rate (error bars represent s.e.m.) of the progeny of hemizygous transgenic males and wild-type females of all transgenic lines with single copy autosomal integrations normalized against the hatching rate of hemizygous transgenic females and wild-type males of the same lines. Experiments were performed in at least two independent generations. The total number of females analysed is summarized in Supplementary Table 2 . Full size image Destabilized I-PpoI distorts the sex ratio towards males To investigate whether the reduction of I-PpoI stability resulted in a dissociation of gamete sex ratio distortion from embryonic toxicity, we determined the larval hatching rate and the number of eggs laid as measures of fertility as well as the adult sex ratio in crosses of transgenic male mosquitoes carrying I-PpoI variants to wild-type female ones ( Supplementary Table 2 ). As a control, transgenic female mosquitoes of each strain were crossed to wild-type male ones. Male mosquitoes of the strain expressing wild-type I-PpoI were sterile as previously observed for the strains gfp I-PpoI-1 and gfp I-PpoI-2 in which I-PpoI was expressed as an eGFP fusion protein [9] . No effect on fertility or the sex ratio was observed in all strains expressing the I-PpoI double-mutant L111A/W124L, which displays the lowest in vitro folded stability ( Fig. 2b,c ) or in strains carrying X-linked transgenes ( Supplementary Fig. 4 ). Significant male-biased sex ratios ranging from 70.2 to 97.4% were observed in the progeny of male mosquitoes carrying the remaining I-PpoI variants ( Fig. 2b ). Some of the strains showed a significant reduction in the number of hatching progeny. Strains carrying I-PpoI variants H106A and W124L suffered a lower impact on their hatching rates than did those carrying the more stable variants L111A and W124A. With the possible exception of variant H106A egg laying rates were generally unaffected and showed little correlation with mRNA expression levels or the I-PpoI variants tested ( Supplementary Fig. 5 ). Notably, strains gfp 111A-2, gfp 124L-2 and gfp 124L-3 combined a high level of male-biased sex distortion (95.0%, 95.5% and 97.4%, respectively) with a fertility rate that did not differ significantly from the controls. Interestingly, these strains also showed the lowest mRNA levels within their respective sets. 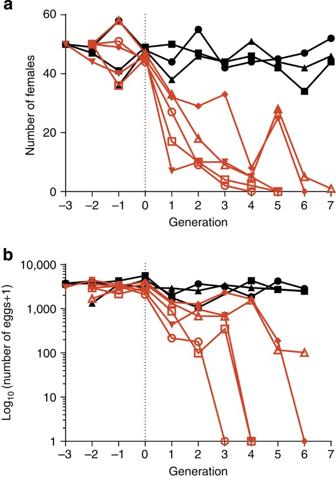Figure 3: Transgenicgfp111A-2 males suppress wild-type mosquito caged populations. Into caged wild-type mosquito populations, initially composed of 50 male and 50 female individuals, hemizygousgfp111A-2 (red lines) or hemizygousgfpI-PpoI-2 control males (black lines) were released starting from generation 0 (dotted line). The release rate of 3X was set relative to the initial number of males in the target population. Shown is the number of adult females in each cage population (a) as well as the number of eggs laid by each of the caged population in that generation (b). We found that, while low rearing temperatures could cause a modest reduction in fertility in gfp 111A-2 male mosquitoes, the sex distortion phenotype remained unaffected at both low (24 °C) and high (32 °C) temperatures ( Supplementary Table 3 ) in all three strains. In addition, we found that the sex distortion phenotype was stably inherited from male mosquitoes to their transgenic sons. For four subsequent generations, transgenic male mosquitoes of gfp 111A-2 fathers showed comparable levels of fertility and male-biased sex ratios in their offsprings ( Supplementary Table 4 ). Finally, we investigated the phenotype of homozygous distorter males since such males would transmit the distorter to all their male progeny resulting in a stronger suppressive effect on target populations. Whereas the addition of an extra copy of the transgene construct in strains gfp 111A-2 and gfp 124L-3 caused a reduction in the hatching rate, it had no effect on the fertility of gfp 124L-2, which showed hemizygous mRNA levels less than half of gfp 124L-3 ( Supplementary Table 5 ). Analysis of individuals with modified X chromosomes We analysed at the molecular and phenotypic levels the small fraction of female offspring of transgenic male mosquitoes and found molecular evidence for both misrepair and copy number variation of the ribosomal gene cluster in these individuals ( Supplementary Fig. 6a,b ). We also observed a significant female-biased sex ratio in the progeny of female survivors crossed to wild-type males suggesting that loss of viability occurs in individuals that had inherited only a damaged X chromosome ( Supplementary Table 6 ). We also investigated whether the X chromosomes of daughters from transgenic males were intrinsically resistant to I-PpoI activity. For this purpose, we utilised daughters of gfp 111A-2 males, carrying paternal ‘modified’ X chromosomes that had been exposed to I-PpoI activity. Females that had also inherited the transgene were crossed to wild-type males. The transgenic male progeny, having a 50% chance of carrying the potentially resistant X chromosome, was then crossed to wild-type females and the sex ratio of individual crosses was recorded. This analysis showed a male bias in the progeny of all males that did not differ significantly from the gfp 111A-2 stock ( Supplementary Fig. 6d ). These experiments suggested that X chromosomes of female survivors are damaged as a result of I-PpoI activity yet remaining susceptible to further cleavage. A stochastic process most likely accounts for the fact that some damaged X chromosomes allow the constitution of functional gametes, resulting in female progeny. Population cage experiments Although the robustness of these traits under variable natural conditions remains to be studied, our findings have important implications for the development of genetic vector control measures. To demonstrate this we performed a set of population cage studies to assess whether the I-PpoI sex distorter strains could suppress wild-type A. gambiae caged populations. We observed in five independent cage experiments that the release of hemizygous gfp 111A-2 males at an over-flooding ratio of 3X was effective in suppressing caged wild-type populations (achieving elimination within six generations in four out of five cages). As expected, the release of sterile ‘control’ males expressing wild-type I-PpoI at the same ratio had no measurable effect on three control populations ( Fig. 3 ) under these experimental conditions. We observed hatching rates averaging below 20% in the terminal generations of these caged populations, indicating that under field conditions the accumulation of X chromosome damage would significantly contribute to the demise of target populations. Figure 3: Transgenic gfp 111A-2 males suppress wild-type mosquito caged populations. Into caged wild-type mosquito populations, initially composed of 50 male and 50 female individuals, hemizygous gfp 111A-2 (red lines) or hemizygous gfp I-PpoI-2 control males (black lines) were released starting from generation 0 (dotted line). The release rate of 3X was set relative to the initial number of males in the target population. Shown is the number of adult females in each cage population ( a ) as well as the number of eggs laid by each of the caged population in that generation ( b ). Full size image As with any other forms of pest control, it is important to consider possible pathways for the evolution of resistance. The universal conservation of the I-PpoI recognition sequence [12] within the multicopy essential 28S rDNA locus of animals makes the rapid selection of target site resistance unlikely. Other rDNA sequences or alternative X-specific sequence repeats could also be targeted—for example, by recently described programmable DNA endonucleases [13] , [14] . Our findings thus suggest a more universal approach towards achieving sex distortion. The introduction of a sex distorter favouring the production of males into a pest population has been predicted to be a highly effective control strategy [3] . Depending on the use of one or multiple autosomal distorter loci the single releases of such males may be at least two orders of magnitude more effective than sterile males and repeated releases 2–70 times more effective than equivalent releases of female-killing alleles [2] . Using a discrete-generation model specifically parameterized with the properties of our transgenic strains, we find the release of single-locus homozygous I-PpoI males to have a greater suppressive effect than equivalent releases of males causing sterility or female-specific lethality and can effectively reduce vector populations at low release ratios ( Supplementary Fig. 7 ). The scaling up of COPAS automated fluorescent larval sorting technology [10] , [15] or the use of conditional expression systems will facilitate the sustained mass releases of these autosomal strains in the field. In addition, the insertion of the I-PpoI transgene on the male sex chromosome may generate a driving Y chromosome that, in theory, could eliminate a natural vector population even when seeded with a very low number of transgenic males [1] , [16] . Engineering of destabilized I-PpoI variants Eleven individual residues were chosen for mutation based upon their location in any of three separate regions of the protein: coordination of structural zinc ions within the protein fold (C41, C100, C105, H110, C125, C132, H134 and C138), formation of the dimer interface (W124) or packing within the hydrophobic core (H106 and L111). Each residue was individually converted into an alanine. Residue W124 was more extensively altered to phenylalanine, leucine or alanine (which correspond to serial reductions in the size of the larger indole side chain) because that residue plays an important role in the packing of the enzyme dimer interface ( Fig. 1b ). All point mutants of I-PpoI and the wild-type were expressed using a bacterial expression plasmid construct. The vector contains the I-PpoI reading frame (amplified from pI3-941 (ref. 17 )) cloned between the Bam HI and Nde I sites within the pET11c [18] plasmid. The 15 point mutations were incorporated into the I-PpoI scaffold, first individually and then in pairwise combinations as described in the text, using a QuikChange II XL Site-Directed Mutagenesis Kit (Stratagene) following the manufacturer’s protocol. The identity of the point mutants were verified using DNA sequencing. Purification of I-PpoI variants Protein expression and purification was performed as previously described [18] . Briefly, each expression construct was transformed into Escherichia coli BL21-CodonPlus (DE3)-competent cells (Promega Biotech). A 5-ml LB starter culture was inoculated with a single colony and grown at 37 °C for 3–4h h, and then added to 1 l of LB media pre-warmed to 37 °C and grown until OD. 600 of ~0.8. Isopropyl β-D-1-thiogalactopyranoside and zinc acetate were then simultaneously added to concentrations of 0.5 and 1.5 mM, respectively, and the culture was moved to 16 °C and allowed to grow for an additional 16 h. Cells were harvested via centrifugation at 4 °C. Pellets were resuspended in 50 ml of 50 mM Tris pH 8, 100 mM NaCl, 5% Glycerol, 1 mM MgCl 2 , 5 mM dithiothreitol and 0.5 mM phenylmethyl sulphonyl fluoride. Cells were lysed via sonication and centrifuged to remove debris. The supernatant was diluted twofold with 50 mM Tris pH 8 and then applied to a 5-ml HiTrap Heparin HP (GE Healthcare) affinity column equilibrated with 50 mM Tris pH 8. A salt gradient was then run from 0 to 0.6 M NaCl under constant buffering conditions. Using this protocol, wild-type I-PpoI eluted at ~0.4 M NaCl. Those point mutants that were soluble eluted within the bounds of the same salt gradient. The proteins were used immediately in subsequent assays described below. Determination of denaturation temperatures and thermal half-lives Purified I-PpoI variants were diluted to concentrations between 10 and 20 μM and exchanged via overnight dialysis into 10 mM potassium phosphate buffer at pH 8. CD data were collected on a Jasco J-815 spectrometer in a 0.1-cm path length cuvette. Initial UV CD wavelength scans (250 –190 nm) were collected for each construct at 20 °C and then at 90 °C; the wavelength where the change in CD signal strength was greatest (206 nm) was then chosen for monitoring during a variable temperature scan. Temperature melts spanning a range from 4 to 95 °C were measured using 2° increments with temperature regulated by a Peltier device. Sample temperature was allowed to equilibrate for 30 s before measurement. Thermal denaturation half-points ( T m values) were determined by curve-fitting using the SpectraManager software supplied by the manufacturer. In subsequent experiments conducted for each construct, enzyme samples at 11.5 μM protein concentration, under the buffer conditions listed above, were set to a single temperature value (30 or 37 °C), and the loss of CD ellipticity signal (monitored at 206 nm wavelength) was followed for 4 h, with measurements taken every 30 s. The average of the first six values (collected between 0 and 3 min) and of the last six values (collected between 237 and 240 min) were used as values corresponding to the beginning and end points of each experiment (that is, t =0 and t =4 h). The protein was then completely unfolded at 95° and an unfolded baseline signal was monitored for 30 min and also averaged. This value was subtracted from the t =0 and t =4 h ellipticity values described above. These values were then converted to fraction unfolded protein, and each construct’s thermal half-life was determined by assuming (i) that unfolding followed a first-order exponential decay (which agreed well with all unfolding curves over the time course of the experiment) and (ii) that the 95 °C average baseline represents 100% unfolded protein. Using this approach, the thermal half-life (‘ t 1/2 ’) was calculated according to where F =fraction folded and t =time. Determination of specific activity Protein activity cleavage assays were performed using a substrate corresponding to a 937-bp polymerase chain reaction (PCR) product that was generated using the pBend3-Ppo plasmid [19] . To create that plasmid, oligonucleotides containing the I-PpoI target site (5′-CTAGATGACTCTCTTAAGGTAGCCAA-3′ and its complement 5′-TCGATTGGCTACCTTAAGAGAGTCAT-3′) were annealed and then ligated into pBend3 (ref. 20 ) between the Sal I and Xba I restriction sites. The DNA substrate contains the I-PpoI target site flanked by 576 and 361 bp, respectively. I-PpoI constructs were diluted to concentrations ranging from 50 to 1,000 nM enzyme in 10 mM Tris pH 7.5, 50 mM NaCl, 0.1 mM EDTA. Samples were then added in a 1:10 v/v ratio into a standard cleavage buffer (2.5 mM CAPS/CHES pH 10, 5 mM NaCl, 0.2 mM dithiothreitol, 1 mM MgCl 2 , 0.01 mg ml −1 bovine serum albumin and 20 nM DNA substrate), corresponding to final enzyme concentrations of 5–100 nM (adjusted for each construct to allow for production of an easily measurable amount of product during the reaction, without completely digesting the substrate). The digests proceeded at room temperature (23±0.5°) for 5 min and were then quenched with 2 × stop buffer (2% SDS, 0.1 M EDTA, 20% glycerol and 0.2% bromophenol blue). The reaction products were separated and visualized using agarose gel electophoresis (2% TAE) and the resulting bands were quantitated using ImageJ. Generation of germline transformation constructs eGFP::I-PpoI was amplified using the common primer GFP-PpoI-F (5′-GAGCTGTACAAGTCCGGACTCAGA-3′) and unique the chimeric primers: Ppo111A-SanDI (5′-CGTTGGGACCCGGGCACCAGTTTCTGCCTTTGTTGTCGTCTAGCGACTCCCA GCATGCGTGCAAGGGATTGTGGCATCG-3′, Ppo124A-SanDI (5′-CGTTGGGACCCGGGCATGCGTTTCTGCCTTTGTTGTCGTCTAGCGACTCCCA GCACAAGTGCAAGGGATTGTGGCATCG-3′), Ppo124L-SanDI (5′-CGTTGGGACCCGGGCATAAGTTTCTGCCTTTGTTGTCGTCTAGCGACTCCCA GCACAAGTGCAAGGGATTGTGGCATCG-3′) and Ppo111A/124L-SanDI (5′-CGTTGGGACCCGGGCATAAGTTTCTGCCTTTGTTGTCGTCTAGCGACTCCCAGCAT GCGTGCAAGGGATTGTGGCATCG-3′) from pBac[3xP3-DsRed]β2-eGFP::I-PpoI (ref. 9 ). Each 0.45-kb product was digested with Bgl II and San DI and ligated back into pBac[3xP3-DsRed]β2-eGFP::PpoI to generate the final transformation constructs. In order to generate pBac[3xP3-DsRed]β2-eGFP(F2A)I-PpoI, we used primers β2-AfeI-F (5′-CCCAGCGCTTAGAGAGCAACGCTCGTGC-3′) and F2A-NLS-R (5′-CAGCTTCAGCAGGTCGAAGTTCAGCGTCTGCTTCACCGGGGCGCGCTTGGCGC GCTTGTACAGCTCGTCC-3′) as well as primers F2A-NLS-F (5′-CTGAACTTCGACCTGCTGAAGCTGGCCGGCGACGTGGAGTCGAACC CGGGCCCTAAGAAGAAGAGGAAGGTGA-3′, which encode the F2A peptide sequence [21] and Ppo124W-SanDI (5′-CCGTTGGGACCCGGGCACCAGTTTCT GCCTTTGTTGTCGTCTAG-3′) to amplify two fragments from pBac[3xP3-DsRed]β2-eGFP::I-PpoI that were used as template for a second PCR performed with the primer pair β2-AfeI-F and Ppo124W-SanDI. The final 1.3-kb Afe I and San DI digested was ligated into pBac[3xP3-DsRed]β2-eGFP::I-PpoI. In order to obtain the constructs pBac[3xP3-DsRed]β2-eGFP(F2A)I-PpoI-111A and pBac[3xP3-DsRed]β2-eGFP(F2A)I-PpoI-111A/124L, a fragment of 1.9 kb was digested from the respective eGFP::PpoI plasmids and moved into pBac[3xP3-DsRed]β2-eGFP(F2A)I-PpoI to replace the original eGFP::I-PpoI sequence. Each construct contains piggyBac inverted repeats and DsRed under the control of the 3xP3 promoter as a germline transformation marker. Generation of transgenic mosquito lines A. gambiae sensu stricto embryos (strain G3, from here on referred to as wild-type) were injected using a Femtojet Express injector and a Narishige 202ND micromanipulator mounted on an inverted microscope (Nikon TE-DH100W) with a mixture of 0.2 μg μl −1 of the selected plasmid and 0.4 μg μl −1 of helper plasmid containing a vasa -driven piggyBac transposase (Eric Marois, unpublished). An average of 375 embryos was injected for each plasmid with a 17.5% of survivors obtained. The hatched larvae were screened for transient expression of the DsRed marker and positives (~54%) crossed to wild-type mosquitoes. The progeny was analysed for DsRed fluorescence. DsRed positives were crossed individually with wild-type mosquitoes to obtain transgenic lines. Transgenic lines originated from a single integration event were selected using inverse PCR and Mendelian inheritance of the transgene scored in the progeny ( Supplementary Table 1 ). Transgenic mosquitoes were analysed on a Nikon inverted microscope (Eclipse TE200) at a wavelength of 488 nm to detect eGFP expression (Filter 535/20 nm emission, 505 nm dichroic) and 563 nm to detect DsRed expression (Filter 630/30 nm emission, 595 nm dichroic). Transgenic lines were named after the I-PpoI variant (the gfp superscript indicates eGFP fusion) they express followed by an identifier digit. All transgenic lines were maintained in a way so that in each generation transgenic females were backcrossed back to G3 wild-type males. Inverse PCR For each line, 500 ng of genomic DNA were digested with 10 units of Sau3AI or HinP1I as separate reactions; 5 μl of each digestion was re-ligated with T4 DNA ligase (Takara) in a final volume of 20 μl, of which 5 μl were subjected to PCR. The piggyBac flanking regions were initially amplified with primers 5F1 (5′-GACGCATGATTATCTTTTACGTGAC-3′) and 5R1 (5′-TGACACTTACCGCATTGACA-3′) for 5′ junctions; or 3F1 (5′-CAACATGACTGTTTTTAAAGTACAAA-3′) and 3R1 (5′-GTCAGAAACAACTTTGGCACATAT-3′) for 3′ junctions, followed by a second inner PCR reaction using primers 5F2 (5′-GCGATGACGAGCTTGTTGGTG-3′) and 5R2 (5′-TCCAAGCGGCGAATGAGATG-3′) or 3F2 (5′-CCTCGATATACAGACCGATAAAAC-3′) and 3R2 (5′-TGCATTTGCCTTTCGCCTTAT-3′) on 5 μl of the first reaction. Insertion sites were sequenced using primers pB-5SEQ (5′-CGCGCTATTTAGAAAGAGAGA-3′) for 5′ junctions and pB-3SEQ (5′-CGATAAAACACATGCGTCAATT-3′) for 3′ junctions. qRT–PCR and western blot analysis Mosquito abdomens were dissected and 10 pairs of testes from each transgenic line were pooled to constitute a biological replicate for total RNA and protein extraction using TRI reagent (Ambion). RNA was reverse-transcribed using Superscript II (Invitrogen) after TURBO DNA-free (Ambion) treatment following the manufacturer’s instructions. Quantitative real-time–PCRs (qRT–PCR) analyses were performed on cDNA using the Fast SYBR-Green master mix on a StepOnePlus system (Applied Biosystems). Ribosomal protein Rpl19 gene was used for normalization. At least two independent biological replicates from independent crosses were subjected to duplicate technical assays. We used primers RPL19Fwd (5′-CCAACTCGCGACAAAACATTC-3′), RPL19Rev (5′-ACCGGCTTCTTGATGATCAGA-3′), eGFP-F (5′-CGGCGTGCAGTGCTTCA-3′) and eGFP-R (5′-CGGCGCGGGTCTTGT-3′). For the western blot analysis, proteins were separated under denaturing conditions (SDS–PAGE) on 4–15% precast gels (Criterion TGX, Bio-Rad) and subsequently transferred to Hybond ECL membranes (Amersham). Immunoblotting was performed with α-GFP Rabbit mAb and α-Tubulin Rabbit mAb (Cell Signalling Technology) at a 1:1,000 dilution and a 1:1,000 α-rabbit IgG HRP-linked secondary antibody (Cell Signalling Technology) using the Pierce SuperSignal West Femto Substrate (Thermo Scientific). Chemiluminescence signals were recorded using a Bio-Rad ChemiDoc XRS+ system and quantified using the Bio-Rad Image Lab software. rDNA analysis Genomic DNA was extracted from females using the Wizard Genomic DNA Purification Kit (Promega). Primers rgDNA-F4 (5′-GTAAGGGAAGTCGGCAAACTGGATCCG-3′) and rgDNA-R4 (5′-GAGGAAGCCCTCCCACCTATGCTGC-3′) were used to amplify the I-PpoI target site within the ribosomal 28S gene using the Phusion HF polymerase (Thermo Scientific). One-fifth of each PCR product was loaded in a 1.5% agarose gel and the remainder purified (Qiagen PCR purification kit) and then digested with 100 units of I-PpoI for 3 h at 37 °C. The reaction was then run in a 1.5% agarose gel after heat inactivation at 65 °C for 15 min. qRT–PCRs were performed using Rpl19 as internal control for normalization and three independent technical replicates for each sample. Primers rgDNA18S-F (5′-CCGTCCAGACTCGCGTCCGTC-3′), rgDNA18S-R (5′-GGGCACCATGAAGCTGGGTCG-3′) and rgDNA5.8S-F (5′-GGCAGGGGATCACTCGGCTCA-3′), rgDNA5.8S-R (5′-CGTCCGATGCGCCATATGCGTT-3′) were used. Crosses and fertility assays To assay fertility and the adult sex ratio, 10 transgenic males were crossed to 10 wild-type females and as a control 10 transgenic females were crossed to 10 wild-type males ( Fig. 2 and Supplementary Table 2 ). In all crosses, mosquitoes were allowed to mate for 5 and 3 days after the blood meal gravid females were placed individually in oviposition cups. The number of eggs laid as well as the number of larvae hatching were counted. The larvae were then pooled and reared to adulthood. The total number of adult male and female mosquitoes from each cross were subsequently counted. Each transgenic line was assayed for at least two consecutive generations. To determine whether the sex distortion phenotype was stably inherited, 10 gfp 111A-2 males were crossed to 10 wild-type females ( Supplementary Table 4 ). Their transgenic sons were backcrossed in the same way for four consecutive generations. The numbers of eggs, larvae hatched as well as the adult sex ratio were determined as described above. To generate homozygote individuals for the analysis of the effect of transgene copy number, 15 transgenic females and 15 transgenic males were crossed and from the offspring approximately 400 L1 larvae were sorted using a ‘COPAS Mosquito’ large particle flow cytometer (Union Biometrica) using a 488-nm solid-state laser and emission filters for the detection of GFP filter (510 nm, band width of 23 nm) and DsRed filter (610 nm, band width of 20 nm). Homozygote and heterozygote larvae were selected and separated according to the intensity of DsRed fluorescence and 20 individuals of each type were crossed to wild-type females ( Supplementary Table 5 ). The numbers of eggs laid and the larval hatching rate were measured as described. Females were allowed to oviposit individually and the progeny of each female was reared to adulthood separately to determine the sex ratio. To study temperature dependence, three different sets of experiments were performed with gfp 111A-2, gfp 124L-2 and wild-type strains reared at 24 °C, the standard 28 and 32 °C (80% humidity) from larval stage L1 ( Supplementary Table 3 ). gfp 111A-2 and gfp 124L-2 males were crossed to wild-type females and transgenic females were crossed to wild-type males as a control. Mosquitoes were mated for 5 days and females were allowed to lay eggs 3 days after a blood meal at standard temperature of 28 °C. The egg laying and hatching rate as well as the adult sex ratio were determined from the progeny of individual females as described. To test for the occurrence of potentially cleavage-resistance X-chromosomes 10 gfp 111A-2 females, originating from crosses between gfp 111A-2 males with wild-type females, were crossed to 10 wild-type males, in two independent experimental replicates. Twenty transgenic males that originated from these crosses (termed gfp 111A-2 mod ) were individually crossed to wild-type females. As positive and negative controls, 20 gfp 111A-2 stock males or 20 gfp 111A-2 stock females were individually crossed to 20 wild-type females or males, respectively ( Supplementary Fig. 6d ). To analyse the female progeny of transgenic males, we crossed 10 gfp 111A-2 males with 10 wild-type females and then crossed, in four batches, 10–15 transgenic female survivors (termed gfp 111A-2 mod ) with 10–15 wild-type males ( Supplementary Table 6 ). As a control, an equal number of stock gfp 111A-2 females were crossed to wild-type males. The egg laying and hatching rate as well as the adult sex ratio were determined from the progeny of individual females as described. Population cage experiments We initially established eight populations of 50 male and 50 female wild-type individuals in population cages (BugDorm-1, Megaview). Each generation mosquitoes were allowed to mate for 5–7 days and then all females were bloodfed on mice. After 3 days, females were allowed to oviposit and the eggs were washed with 2% household bleach (in water) followed by water on a round filter paper (Whatman, 125 mm). High-resolution images of these filter papers were taken and used to automatically count all eggs using the Anopheles Eggcounter software [22] . To approximate a natural population growth rate of approximately nine females produced per female we applied a mortality rate of 50% at the egg stage. This was performed by cutting the filter paper containing eggs in half or by counting and selecting eggs manually when there were fewer than ~200 eggs. The remaining eggs were hatched and a maximum of 110 L1 larvae selected at random and moved to a new tray to be reared to the pupal stage at which all individuals were manually sexed and males and females were allowed to emerge in separate holding cages. After 48 h males and females as well as 150 release males (during the intervention phase) were introduced into a new cage to establish the next generation. The rationale for this approach is as follows: we established in the initial generations before releases that females laid an average of 2,815 eggs per cage or ~56.3 eggs per per female under these conditions. Using COPAS sorting we counted all larvae and determined a hatching rate of 68.4% under these conditions. Around 90% of larvae reared under these conditions reached the adult stage. Hemizygous release males (either gfp 111A-2 males or gfp I-PpoI-2 males for sterile control releases) were reared in separate trays under identical conditions alongside the main populations but were COPAS-sorted at the L1 stage for the presence of the fluorescent transgene. Discrete generations model of mosquito dynamics The dynamics of the mosquito population is described by a discrete-generation model. Each adult female produces a number f of progeny per generation. This progeny survives to adulthood with a probability P L that declines with the density of larvae (L): P L = θ L × F (L), where θ L is the probability of surviving through the larval stage at very low density and F (L) characterizes the density-dependent survival arising from the competition among larvae and following a Beverton–Holt equation . The recurrence for the number of female adults ( A t ) is therefore: Parameterisation: f =130.1, θ L =0.076 and α =500,000. In the absence of control, equation (2) set for equilibrium provides the equilibrium density value: . We investigate the equilibrium density of vectors as a function of the number of males released per generation for each control strategy. Solutions were derived either analytically (for SIT and RIDL) or numerically (for autosomal X-shredder) allowing to compare the thresholds of minimal release size to eliminate the target mosquito population for the different strategies. Modelled control strategies Releases of intervention males into the population result in a genetic and phenotypic diversity that is incorporated into the model by distinguishing groups of individuals with identical genotypes and thus identical life-history traits. In both models, females are assumed to mate once in their life, on the first day they emerge, with a male chosen at random from the entire adult population. We characterize adult females according to their genotype and that of their mate: A ij is a female of genotype i and fertility f i that mated a male of genotype j , . Each of these matings gives rise to a specific set genotypes in the progeny. Individuals carrying autosomal sex ratio distorters are indexed by whether they have 0, 1 or 2 autosomal copies of the distorter transgene, which is inherited in a Mendelian manner. At male meiosis, these alleles induce shredding of the X chromosome and distort to m x the proportion of gametes that inherit the Y chromosome. We consider two types of releases: males being either heterozygous or homozygous carriers of the distorter transgene. Males carrying Y-linked sex ratio distorters are indexed by whether they carry the distorter-bearing Y or not. The construct induces X shredding and is transmitted along the Y to a proportion m x of sperm. By mating with wild females sterile males (SIT strategy) prevent the generation of viable progeny and reduce the recruitment of the next generation. Individuals carrying a dominant late-acting lethal gene (RIDL strategy) are indexed by whether they have 0, 1 or 2 RIDL alleles. These dominant alleles induce the death of mosquitoes (either in both sexes ‘bisexual form’ or in females only ‘female-specific form’) at the end of the larval stage. How to cite this article: Galizi, R. et al . A synthetic sex ratio distortion system for the control of the human malaria mosquito. Nat. Commun. 5:3977 doi: 10.1038/ncomms4977 (2014).